Nanoscale imaging and spontaneous emission control with a single nano-positioned quantum dot Plasmonic nanostructures confine light on the nanoscale, enabling ultra-compact optical devices that exhibit strong light–matter interactions. Quantum dots are ideal for probing plasmonic devices because of their nanoscopic size and desirable emission properties. However, probing with single quantum dots has remained challenging because their small size also makes them difficult to manipulate. Here we demonstrate the use of quantum dots as on-demand probes for imaging plasmonic nanostructures, as well as for realizing spontaneous emission control at the single emitter level with nanoscale spatial accuracy. A single quantum dot is positioned with microfluidic flow control to probe the local density of optical states of a silver nanowire, achieving 12 nm imaging accuracy. The high spatial accuracy of this scanning technique enables a new method for spontaneous emission control where interference of counter-propagating surface plasmon polaritons results in spatial oscillations of the quantum dot lifetime as it is positioned along the wire axis. Controlled interactions between nano-emitters and plasmonic nanostructures are important for a broad range of applications in photonics and quantum optics. Plasmonic nanostructures localize electromagnetic fields to nanometre dimensions in the form of surface plasmon polariton (SPP) waves. Accurate placement of nano-emitters in the high-field regions of SPP modes can improve the efficiency and directionality of light emitters [1] , [2] , provide large nonlinear optical effects at low light levels [3] , [4] , [5] , enhance sensing capabilities [6] , [7] and enable the development of lump-element nanophotonic circuits [8] as well as quantum optical circuits for quantum networking [4] , [9] . Nano-emitters can also serve as nearly ideal localized excitation sources that can be used to probe electromagnetic properties of plasmonic nanostructures, such as the local density of optical states (LDOS), with high spatial resolution [10] . A variety of methods have been applied for sub-wavelength probing of plasmonic structures. Near-field scanning optical microscopy utilizes a tapered tip to probe the LDOS [11] , [12] , [13] , [14] , [15] , [16] . This tapered probe, however, can add unwanted distortion to the image [10] , [17] , [18] . Other imaging techniques, such as electron energy-loss spectroscopy [19] and cathodoluminescence imaging spectroscopy [20] , [21] , enable the study of plasmonic mode structures with nanometric precision by using a tightly focused electron beam. However, these techniques typically require high vacuum and an electron beam that has been accelerated at high voltage, which has limited their applicability. An ideal probe for nanoscale electromagnetic imaging is a single, isolated, point-like dipole emitter, which provides high spatial resolution with minimal distortion of the LDOS [10] . Additionally, the strong back-action of the plasmonic nanostructure on the emitter can enhance or suppress spontaneous emission. This back-action provides an effective method for performing spontaneous emission control [22] , [23] , forming the basis for novel light sources [2] and quantum circuits [4] . Methods that incorporate either single emitters [24] , [25] or ensembles of emitters [23] , [26] on a scanning tapered probe have been demonstrated for both near-field imaging and spontaneous emission control, but these techniques have so far been limited to an imaging resolution of about 100 nm. Mechanical dragging of diamond nanocrystals in the vicinity of plasmonic structures using scanning-probe manipulators has also been demonstrated [27] , [28] , but to date this method has only provided sparse sampling of the electromagnetic mode with too few data points to reconstruct an accurate image. Three-dimensional manipulation of 75-nm diamond nanocrystals by optical trapping has also been reported recently and used to image the LDOS of dielectric waveguides [29] , but the extension of this approach to plasmonic structures is challenging because the field typically decays on a length scale that is on the order of the size of the nanocrystal. Random diffusion of fluorescent molecules has also been used to image plasmonic hot spots, achieving spatial imaging accuracy as fine as 1.2 nm (ref. 30 ). However, this procedure is entirely stochastic and cannot be used to probe a desired location or target on demand. Semiconductor quantum dots (QDs) are ideal nano-emitters for local probing and excitation of plasmonic nanostructures. QDs are bright and highly efficient room-temperature light sources with a stable, narrow and tunable emission spectrum [31] . They also exhibit single-photon emission, making them potential candidates for quantum devices [32] . Additionally, owing to their nanometric size, QDs can act as sensitive probes for studying the electromagnetic properties of plasmonic nanostructures with high spatial accuracy. However, the application of QDs as nanoscale probes has been challenging. Their small size makes them difficult to manipulate using standard approaches such as optical trapping [33] . Although optical trapping of single QDs has been demonstrated [34] , the spatial accuracy of this trapping procedure has not been reported and the positioning accuracy that can be achieved with this approach remains unclear. Additionally, optical trapping forces are not selective, which can result in many particles getting caught in a single trap over a short timescale. Alternate methods that utilize tapered probes with single QDs attached to the tip [35] or, conversely, scan an attached sample over a single QD immobilized on a surface [36] , have been reported. However, these approaches have been largely limited by QD blinking and bleaching, which significantly distort the acquired image. In this work, we demonstrate that a single QD can be used as a nanoprobe for imaging plasmonic nanostructures and for spontaneous emission control with high spatial accuracy. Specifically, we use a single QD to image the LDOS of a silver nanowire (AgNW). The QD is deterministically positioned at desired locations adjacent to the AgNW by actuating flow in a microfluidic device through electroosmosis [37] , thereby moving the QD via viscous drag [38] , [39] . Using this approach, we image the LDOS with a spatial accuracy as fine as 12 nm. Furthermore, we utilize the back-action of the AgNW on the QD to perform spatially resolved spontaneous emission control with nanoscale accuracy. We demonstrate control of the QD lifetime by placing it in regions with different magnitudes of the LDOS. The high spatial accuracy of our approach reveals oscillations in the QD spontaneous emission rate, as it is positioned along the wire axis. These oscillations are the signature of direct coupling to surface plasmon modes induced by interference between counter-propagating surface plasmon waves. The ability to control light–matter interactions at these length scales is crucial for optimizing interactions between single emitters and surface plasmons, and has an important role in the study of quantum optics in plasmonic structures as well as in the development of nanoscale quantum devices [4] . Description of imaging approach Our imaging approach relies on the strong electromagnetic interactions between the QD and the SPP mode of the wire. When a QD is positioned near an AgNW, energy from the photoexcited QD is transferred to the wire’s SPP mode through an electric dipole interaction [22] . The rate of energy decay of an isotropic emitter into the guided SPP mode of the AgNW is given by Fermi’s Golden Rule where D ( ω ) is the spectral density of electromagnetic modes, E ( r , ω ) is the electric field operator for the AgNW mode and μ is the transition dipole moment of the emitter [40] . Although QDs can exhibit polarized light emission and are therefore not completely isotropic [41] , rotational Brownian motion in the fluid averages out orientational effects on a timescale that is much faster than the data integration time ( Supplementary Fig. S1 ), enabling the QD to behave as an effectively isotropic emitter. The spontaneous emission rate is often expressed in terms of the LDOS defined as [42] : where k = ω / c . Thus, γ nw is proportional to the LDOS, and provides a direct measure of the local field intensity of the AgNW mode at the location of the emitter. In our experiment, this rate is measured in two independent ways: by monitoring the radiated light intensity from the wire end and by directly measuring the QD lifetime as a function of position. These two observables provide mutually complementary approaches for studying the electromagnetic properties of the wire. Experimental procedure An optical image of the microfluidic device used to position QDs is shown in Fig. 1a . Four microfluidic channels intersect at the control region, where QD manipulation occurs (the dashed circle). 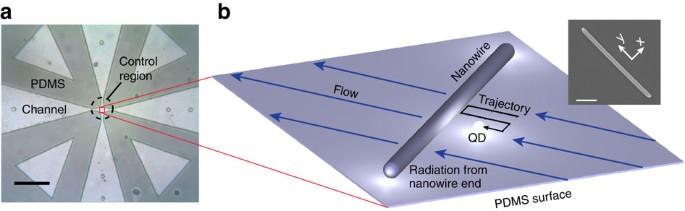Figure 1: Near-field probing with a single QD. (a) Optical image of the microfluidic crossed-channel device. Flow in the centre control region (dashed circle) is manipulated in two dimensions by four external electrodes (not shown). Scale bar, 500 μm. (b) Schematic of the positioning and imaging technique. A single QD is driven along a trajectory close to the wire by flow control. The coupling between the QD and AgNW is measured either by the radiated intensity from the wire ends or by QD lifetime measurements. The inset shows a scanning electron microscopy image of a typical AgNW used in our experiments (scale bar, 1 μm). Thex–ycoordinate system is defined relative to the orientation of the AgNW, as illustrated in the inset. Figure 1b illustrates the probing procedure for an AgNW. Within the control region, a single QD is selected and driven along a trajectory that samples the LDOS of the wire at a desired set of locations. AgNWs with an average diameter of 100 nm and an average length of 4 μm (scanning electron microscopy image in Fig. 1b inset) are deposited on the polydimethylsiloxane (PDMS) surface of the control region. The channels are filled with fluid containing QDs that are confined to a thin sheath along the surface by the fluid chemistry [39] . Within this sheath, single QDs are manipulated to nanometric accuracy using flow control. The deposited AgNW acts as an obstacle for the QDs ( Supplementary Movie 1 ), indicating that the QDs are constrained to be within 100 nm of the surface (the diameter of the AgNW). The QD fluorescence signal is collected using a confocal micro-photoluminescence system [38] , [39] , and 25% of the emission is sent to a CCD camera for tracking. The remaining 75% of the emission is sent to an avalanche photodiode (APD) for performing lifetime measurements. Each detection event from the APD is saved with a time stamp that is synchronized to the camera frame acquisition rate. Details of the fluid composition, experimental set-up and nanowire synthesis are provided in the Methods section. Figure 1: Near-field probing with a single QD. ( a ) Optical image of the microfluidic crossed-channel device. Flow in the centre control region (dashed circle) is manipulated in two dimensions by four external electrodes (not shown). Scale bar, 500 μm. ( b ) Schematic of the positioning and imaging technique. A single QD is driven along a trajectory close to the wire by flow control. The coupling between the QD and AgNW is measured either by the radiated intensity from the wire ends or by QD lifetime measurements. The inset shows a scanning electron microscopy image of a typical AgNW used in our experiments (scale bar, 1 μm). The x – y coordinate system is defined relative to the orientation of the AgNW, as illustrated in the inset. Full size image QD positions are tracked with sub-wavelength accuracy by fitting the imaged diffraction spot to a Gaussian point-spread function. The spatial accuracy of the tracking algorithm is limited by system vision noise, which includes a combination of camera read noise, multiplication noise and shot noise. We determine the tracking accuracy by monitoring an immobilized QD on a glass surface for 1 min. The measured QD positions are plotted as red data in Fig. 2a . The red bars in Fig. 2b plot a histogram of the measured QD position along x and y coordinates respectively. The solid yellow line represents a Gaussian fit where the standard deviation (s.d.) is used to determine a tracking accuracy of σ tr =12±1 (11±1) nm along the x ( y ) directions. 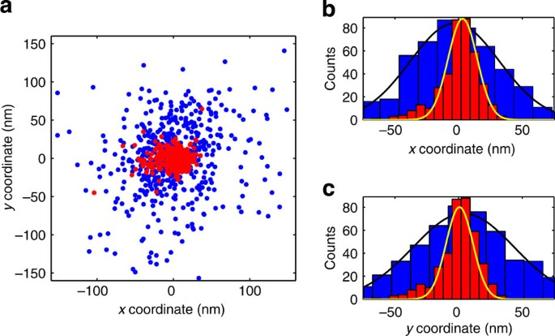Figure 2: QD tracking and positioning accuracy. (a) Scatter plots of the measured positions of a QD over the course of 1 min. Red data points correspond to a QD that is immobilized, while blue data points correspond to a QD that is held in place by flow control. (b,c) Histograms of thexandycoordinate corresponding to data from panela. Red bars are the histogram for an immobilized QD, while blue bars are the histogram for a positioned QD. The yellow solid line is a Gaussian fit for an immobilized QD showing a measure s.d. of 12±1 (11±1) nm along thex(y) coordinate. The black solid line is a Gaussian fit for the positioned QD with s.d. of 36±2 (40±2) nm for thex(y) coordinate. Figure 2: QD tracking and positioning accuracy. ( a ) Scatter plots of the measured positions of a QD over the course of 1 min. Red data points correspond to a QD that is immobilized, while blue data points correspond to a QD that is held in place by flow control. ( b , c ) Histograms of the x and y coordinate corresponding to data from panel a . Red bars are the histogram for an immobilized QD, while blue bars are the histogram for a positioned QD. The yellow solid line is a Gaussian fit for an immobilized QD showing a measure s.d. of 12±1 (11±1) nm along the x ( y ) coordinate. The black solid line is a Gaussian fit for the positioned QD with s.d. of 36±2 (40±2) nm for the x ( y ) coordinate. Full size image Nanoscale positioning accuracy is achieved by employing vision-based feedback control that creates corrective flows to position the QD at a desired location. The positioning accuracy is measured by monitoring a QD that is held in place by flow control for 1 min. The measured QD positions are plotted as blue data points in Fig. 2a . The blue bars in Fig. 2b are a histogram of these measurements, while the black solid line is a Gaussian fit where the s.d. determines a positioning accuracy of σ p =34±3 (39±3) nm along the x ( y ) directions. These numbers were corrected for noise in the tracking algorithm using the relation , where σ is the total measured position fluctuations. The high positioning accuracy ensures that we can deterministically probe the wire mode at a desired location on demand with nanometric accuracy. It is important to note that the positioning accuracy does not limit the spatial imaging accuracy of the system, as the position of the QD is known to a higher accuracy than it can be controlled. 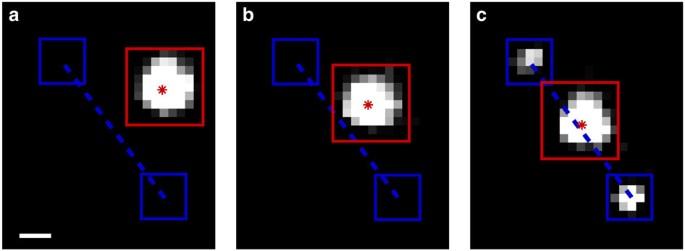Figure 3: Coupling a QD to an AgNW. (a–c) A series of images showing coupling of the QD to the AgNW as the QD is moved closer to the wire. The scale bar is 500 nm and intensities are plotted on a logarithmic scale. The red and blue boxes show the image integration region used to calculate the radiation intensities and positions of the QD and the wire ends, respectively. The measured location of the QD is labeled with a red star and the axis of the AgNW is labelled with a blue dashed line. Figure 3a–c shows a series of images of a single QD being moved progressively closer to an AgNW ( Supplementary Movie 2 ). When the QD is in close proximity to the wire, light radiates from the wire ends ( Fig. 3c ). This radiation arises from direct dipolar coupling of the QD excitation to the waveguided SPP mode. The extraction efficiency of the QD excitation into the AgNW mode is given by η ex = γ nw / γ , where γ is the total decay rate of the QD due to all radiative and non-radiative decay channels and γ nw is defined in equation (1). In the limit in which γ is dominated by free-space modes, the efficiency is proportional to the LDOS at the location of the emitter. Therefore, by simultaneously monitoring the QD position and the radiated intensity from the wire end, we can construct an image of the LDOS. In addition, we measure the LDOS by directly measuring the QD radiative lifetime [23] . Such direct lifetime measurements have the advantage that they are independent of sample geometry, as they do not rely on monitoring the AgNW end radiation. Thus, in contrast to measurements that monitor the distal end of a wire, lifetime imaging can be applied to objects that are sub-wavelength in all three dimensions, such as metallic nanospheres and nanorods. Figure 3: Coupling a QD to an AgNW. ( a – c ) A series of images showing coupling of the QD to the AgNW as the QD is moved closer to the wire. The scale bar is 500 nm and intensities are plotted on a logarithmic scale. The red and blue boxes show the image integration region used to calculate the radiation intensities and positions of the QD and the wire ends, respectively. The measured location of the QD is labeled with a red star and the axis of the AgNW is labelled with a blue dashed line. Full size image QD probing was performed at various locations along the middle and end of the AgNW. The QD trajectory was selected to maximize data sampling near the wire surface ( Supplementary Fig. S2 ). A significant challenge of probing with QDs is that they blink [43] , which leads to emission intensity fluctuations that complicate the interpretation of the radiated intensity from the wire end. Our imaging approach offers a convenient solution to this problem because it enables the simultaneous measurement of the intensity radiated both from the wire end and directly from the QD. The direct radiation from the QD is used to normalize for QD blinking and local field enhancement of the pump. The QD emission and the AgNW-radiated intensity are measured by summing the pixels within their respective windows ( Fig. 3a–c ). We define the normalized coupled intensity as: where and are the intensities of the ( n , m ) th and ( p , q ) th pixels within the AgNW and QD windows respectively, while I BKG is the average pixel background intensity. The background level is calculated by averaging pixels sufficiently far away from the AgNW and the QD. The value of is proportional to the coupling efficiency η , and thus to the LDOS of the nanowire. 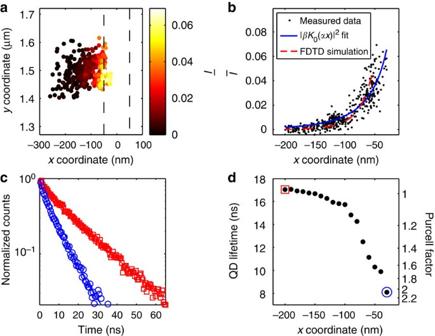Figure 4: Probing the LDOS profile near the middle of the AgNW. (a)as a function of position near the middle of the wire. The dashed region indicates the assumed location of the AgNW surface. (b)as a function of distance from the wire axis (xcoordinate) using data from panela. The blue line indicates the best fit to a modified Bessel function. The red dotted line is an FDTD simulation of the AgNW evanescent field. The simulation result was fit to the data using an overall scaling factor. (c) Radiative decay of the QD at 200 nm (red squares) and 30 nm (blue circles) distance from the AgNW axis with lifetime fits of 17 and 8 ns, respectively. (d) QD lifetime as a function ofxposition. The secondy-axis denotes the Purcell factor corresponding to the measured lifetimes. Coloured markers indicate the data points used for panelc. Probing the side of an AgNW Figure 4a is a scatter plot of as a function of QD position when the QD was positioned near the midpoint of the AgNW. The dashed lines represent the location of the AgNW surface which is assumed to be 50 nm from the wire axis (the typical radius of the wires used in this work). The wire orientation and length were determined by tracking the diffraction spots of the radiated light from the wire ends (blue boxes in Fig. 3c ) using the same algorithm used to track the QD. The data points are plotted relative to the measured wire location with the y -direction aligned along the wire axis and the x -direction corresponding to distance from the wire axis, as indicated in the inset of Fig. 1b , with the origin placed at the lower end of the wire. We note that different locations along the y coordinate may experience different propagation losses to the wire end, which could cause a small distortion of the image. However, the absorption length of an AgNW was measured to be 4.7 μm ( Supplementary Fig. S3 and Methods ), which is much longer than the 200 nm scanning distance. Thus, propagation losses are expected to have only a minimal effect on the data. Figure 4: Probing the LDOS profile near the middle of the AgNW. ( a ) as a function of position near the middle of the wire. The dashed region indicates the assumed location of the AgNW surface. ( b ) as a function of distance from the wire axis ( x coordinate) using data from panel a . The blue line indicates the best fit to a modified Bessel function. The red dotted line is an FDTD simulation of the AgNW evanescent field. The simulation result was fit to the data using an overall scaling factor. ( c ) Radiative decay of the QD at 200 nm (red squares) and 30 nm (blue circles) distance from the AgNW axis with lifetime fits of 17 and 8 ns, respectively. ( d ) QD lifetime as a function of x position. The second y -axis denotes the Purcell factor corresponding to the measured lifetimes. Coloured markers indicate the data points used for panel c . Full size image Figure 4b shows as a function of radial distance from the wire axis, which is seen to increase as the QD approaches the wire surface. For a cylindrically symmetric AgNW, the evanescent field from the surface is predicted to follow a Bessel-function decay [44] . The data are therefore fit to a function of the form where is the zeroeth-order modified Bessel function, x is the distance from the AgNW axis, and α and β are fitting parameters (calculated from the fit to be 0.006 nm −1 and 0.142, respectively). The solid blue line in Fig. 4b is the Bessel-function fit and the red dashed line corresponds to the AgNW evanescent field as calculated using finite-difference time-domain (FDTD) simulation (see Methods). The FDTD solution was multiplied by a constant to provide the best fit to the data. Both the analytical and numerical solutions show good agreement with the measured LDOS profile. The measurements in Fig. 4b can be used to infer the spatial imaging accuracy. This accuracy is determined by calculating the root-mean-square (r.m.s.) deviation in the measured positions of the QD relative to the position predicted by the Bessel-function fit. The rms deviation provides an upper bound on the spatial imaging accuracy, as derived in the Supplementary Methods (see also Supplementary Fig. S4 ). Using this approach, the spatial imaging accuracy was determined to be 12 nm, which is consistent with the 12±1 nm tracking accuracy calculated previously by observing an immobilized QD, indicating that the spatial imaging accuracy is primarily limited by vision noise. The spontaneous emission lifetime of the QD was measured using the APD, while the camera simultaneously measured the QD position. Figure 4c shows two time-resolved fluorescence measurements obtained by collecting photon events detected when the QD was at radial distances of 200±12 nm (red squares) and 30±12 nm (blue circles) from the wire axis, respectively. A biexponential fit was used to determine the QD’s lifetime [45] , yielding values of 17 and 8 ns for the two distances, respectively. This reduction in lifetime at short distance is consistent with previous measurements of QDs coupled to nanowires [22] . Figure 4d plots the QD lifetime as a function of position. Each lifetime was calculated by grouping all photon events in which the QD was within a ±12 nm window from the specified radial distance. The positional dependence of the lifetime mirrors the intensity of the emission from the wire end, demonstrating a clear agreement between the two methods, as well as the ability to perform spontaneous emission control by localizing the QD near the wire surface. The colour scale in Fig. 4d is labelled both in units of raw lifetime (left labels) and Purcell factor (right labels), which is defined as , where is the emission rate of the QD far from the AgNW and γ is the measured decay rate. 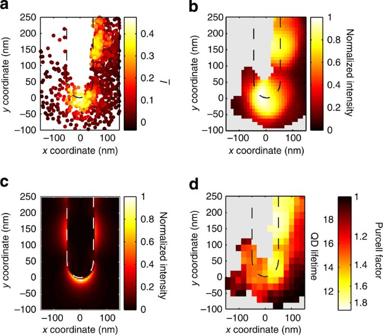Figure 5: Probing the tip of an AgNW. (a) Scatter plot of measured positions and intensities near the end of the AgNW. The colour of each data point corresponds to. The dashed region indicates the location of the AgNW. (b) Reconstructed image using a Gaussian-weighted average. The image intensity is normalized by its maximum. (c) FDTD simulation of the AgNW mode profile showing an enhancement at the tip (also normalized by its maximum). (d) Image of the measured QD lifetime as a function of position. The colour scale is labelled with both lifetime and Purcell factor. Probing the tip of an AgNW Figure 5a is a scatter plot of data recorded when a QD was scanned near one end of the AgNW, while the intensity was monitored at the opposite end. Probing the AgNW tip required several minutes of QD scanning. Over this time span, sample drift can be appreciable, potentially creating image distortion. To account for sample drift, the QD position was measured relative to the wire end that was tracked throughout the experiment. The ability to correct for drift represents an important practical advantage of this approach, enabling us to acquire images over long periods without distortion. Figure 5: Probing the tip of an AgNW. ( a ) Scatter plot of measured positions and intensities near the end of the AgNW. The colour of each data point corresponds to . The dashed region indicates the location of the AgNW. ( b ) Reconstructed image using a Gaussian-weighted average. The image intensity is normalized by its maximum. ( c ) FDTD simulation of the AgNW mode profile showing an enhancement at the tip (also normalized by its maximum). ( d ) Image of the measured QD lifetime as a function of position. The colour scale is labelled with both lifetime and Purcell factor. Full size image The raw data presented in Fig. 5a can be used to construct an image of the LDOS. The value of each pixel in the image is found by taking a Gaussian-weighted spatial average of the raw data. The Gaussian is centred at the location of the pixel and the s.d. is set to 33 nm, corresponding to the rms-combined spatial accuracy of the QD (12 nm) and the tracked AgNW end (30 nm) ( Supplementary Fig. S5 ). The reduced spatial accuracy at the wire ends is attributed to the fact that their emission is much dimmer than the direct QD emission, as can be seen in Fig. 3c . The additional error incurred by tracking the wire end is not fundamental to the imaging procedure and could be largely removed by using brighter tracking objects to monitor the drift. The resulting two-dimensional image is shown in Fig. 5b . Comparison of the measured LDOS profile with the calculated mode obtained from FDTD simulations ( Fig. 5c ) shows good agreement. Figure 5d plots the measured QD lifetime in the region around the AgNW tip. Each lifetime measurement was obtained by combining all photon events for which the QD was within a 33-nm radius of the centre pixel location. The measured lifetime exhibits good agreement with the results obtained from measuring the intensity of the wire end. Spatial oscillation of the LDOS due to interference In addition to the high field intensity at the wire end, the data in Fig. 5 suggest the presence of an oscillatory mode structure along the sides of the AgNW. To examine this mode structure in more detail, the LDOS was probed along a 500-nm region at one end of a wire. The measurement results for are shown in Fig. 6a , where position is once again plotted relative to the wire end to compensate for drift. In this measurement, the QD was positioned as closely as possible to the wire surface. Under these conditions, most of the QD positions were measured within the dashed AgNW region. Data points located within this region are attributed to the QD being pushed slightly onto the top of the wire, which does not act as a perfect obstacle. 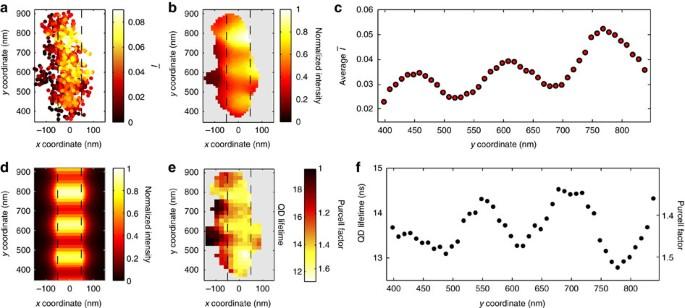Figure 6: SPP wave interference along an AgNW. (a) Scatter plot of the measured QD positions near the end of the wire. The colour of each data point corresponds to the value ofmeasured at each location. The dashed region indicates the location of the AgNW. (b) Reconstructed image using a Gaussian-weighted average. The image intensity is normalized by its maximum. (c) Plot of an averaged value ofas a function of position along the wire. (d) FDTD simulation of the field intensity standing-wave pattern along the side of the AgNW (normalized by its maximum), with the profile within the dashed wire region corresponding to the field immediately outside the wire. (e) Image of the measured QD lifetime as a function of position. The colour scale is labelled with both lifetime and Purcell factor. (f) Plot of QD lifetime measured along the length of the AgNW. Figure 6: SPP wave interference along an AgNW. ( a ) Scatter plot of the measured QD positions near the end of the wire. The colour of each data point corresponds to the value of measured at each location. The dashed region indicates the location of the AgNW. ( b ) Reconstructed image using a Gaussian-weighted average. The image intensity is normalized by its maximum. ( c ) Plot of an averaged value of as a function of position along the wire. ( d ) FDTD simulation of the field intensity standing-wave pattern along the side of the AgNW (normalized by its maximum), with the profile within the dashed wire region corresponding to the field immediately outside the wire. ( e ) Image of the measured QD lifetime as a function of position. The colour scale is labelled with both lifetime and Purcell factor. ( f ) Plot of QD lifetime measured along the length of the AgNW. Full size image A periodic pattern is observed in the scatter plot along the length of the AgNW. These oscillatory fringes arise from interference between the QD emission component coupled to the forward propagating SPP wave and the backward propagating wave that is reflected from the wire end [46] . The oscillatory pattern is more readily observed in the Gaussian image reconstruction ( Fig. 6b ). Figure 6c shows plotted as a function of the y coordinate, where each data point is averaged over a ±33 nm window centred at the y coordinate. Averaging is performed only for points that are within 50 nm of the wire axis. By measuring the peak-to-peak distance from Fig. 6c , we determine the wavelength of the SPP mode to be 320 nm, which is consistent with the 329 nm wavelength calculated from FDTD simulations. The simulated FDTD field profile is displayed in Fig. 6d and exhibits good qualitative agreement with the measured data. The spatial dependence of the QD lifetime along the AgNW is shown in Fig. 6e . The lifetime in a given pixel was measured by consolidating all photon count events when the QD was within 33 nm of the centre location of the pixel. Figure 6f plots the QD lifetime when photon counts were combined using the same spatial window used to obtain Fig. 6c . A clear oscillation in the QD lifetime is observed, mirroring the oscillations in intensity from the wire end. The QD lifetime oscillation is caused by interference between the spontaneous emission components of the forward and backward propagating SPP waves. This mechanism for modifying the spontaneous emission provides an important means of controlling and optimizing light–matter interactions between quantum emitters and nanophotonic structures. The oscillations in Fig. 6 result from the interference between the forward propagating SPP wave and the backward wave that reflects from the near end of the AgNW. Interference will occur so long as the length difference between the two paths of the SPP waves is within the coherence length of the optical field, which can be determined from the measured emission spectrum of a single QD. This measurement was performed using a grating spectrometer ( Supplementary Fig. S6 ). The spectral bandwidth of the QD emission, in units of free space wavelength, was determined to be nm centred at a wavelength of nm, which agrees well with other measured results [47] , [48] . The coherence length of the field propagating in the AgNW can be calculated directly from the measured spectral bandwidth using the relation [49] where =320 nm is the measured wavelength of the SPP mode and . From the measured QD emission bandwidth and wavelength of the SPP mode, the coherence length is calculated to be 1.89 μm, which is long enough to observe good interference at a distance of up to 944 nm away from the AgNW end. Thus, the relatively narrow emission bandwidth of QDs makes them ideal candidates for studying interference and coherent optical effects in plasmonic nanostructures. It should be noted that other nanoscopic emitters, such as fluorescent molecules and nitrogen vacancy centres in nanodiamonds, can have much broader room-temperature emission linewidths [50] , [51] , sometimes exceeding 100 nm. These broad linewidths result in a significantly reduced coherence length, making it more difficult to probe interference effects without spectral filtering, which would result in a large reduction of measured signal. In conclusion, we have demonstrated a technique for both nanoscale imaging of the LDOS of a AgNW and spontaneous emission control using a single nano-manipulated QD. These results enable on-demand control of light–matter interactions and provide a highly flexible method to optimize coupling between single quantum emitters and nanophotonic structures. Additionally, the probing method that we have presented could also find applications in the study of other nanoscale phenomena such as Förster resonance energy transfer [26] and local electric field sensing [52] . We note that the demonstrated probing technique is highly robust to emitter degradation and photobleaching [48] . If the probe emitter degrades, it can be discarded and a replacement can be selected from the ensemble to continue the scan seamlessly, enabling image acquisition over long integration times. Combining this probing scheme with precision placement and immobilization of individually chosen QDs [39] would enable deterministic and optimized assembly of active quantum emitter and plasmonic structures for development of nanoelectronic devices [8] and quantum optical circuits [4] . Fluid composition The control fluid was composed of 45–48% by volume ethoxylated-15 trimethylolpropane triacrylate resin (SR-9035, Sartomer), 1.25–1.4 wt% rheology modifier (Acrysol RM-825, Rohm and Haas Co.) [53] , 0.15–0.3% of a zwitterionic betaine surfactant [54] and CdSe/ZnS core-shell QDs (Ocean NanoTech, Carboxylic Acid, 620 nm) in deionized water. The triacrylate resin causes the fluid sheath to form. The surfactant was introduced to improve electroosmotic actuation on the PDMS surface, while the rheology modifier was used to reduce Brownian motion and inhibit unwanted adhesion of the QDs to surfaces. Experimental set-up The microfluidic device was composed of a moulded PDMS cross pattern placed on top of a glass coverslip. The resulting channel was 5 μm in height with a control region that was ~100 μm in diameter. The QDs were excited simultaneously by a 532-nm continuous wave laser at an intensity of 250 W cm −2 and a 405-nm pulsed laser with a 10-MHz repetition rate at 35 W cm −2 . A fraction (25%) of the QD emission was imaged using an EMCCD camera (Hamamatsu C9100-13) operating at 10 Hz frame rate, while the remaining signal was focused onto an APD (PerkinElmer SPCM-AQR) for time-resolved lifetime measurements. Data were analysed using a time correlation single-photon-counting module (PicoQuant PicoHarp300) that synchronizes photon events with camera frames. Synthesis of AgNWs AgNWs were synthesized by reducing AgNO 3 with ethylene glycol (EG) [55] . In a typical synthesis, 5 ml of EG (Fisher Scientific) was placed in a 50-ml round-bottom flask equipped with a condenser, a thermometer and a magnetic stirring bar. After the EG was heated to 160 °C in an oil bath, 0.5 ml of PtCl 2 (Aldrich, 1.5 × 10 −4 M in EG) was injected into the solution to synthesize 1–5 nm precursor nanoparticles. After 4 min, 2.5 ml of AgNO 3 (Aldrich, 0.12 M in EG) and 5 ml of poly(vinyl pyrrolidone), (Mw≈40,000, City Chemical LLC, 0.36 M in EG) were added simultaneously over 6 min with an accompanying colour change from yellow to yellowish grey. When the AgNO 3 had been completely reduced by EG for 60 min, the solution was cooled to room temperature. To remove the remaining EG, poly(vinyl pyrrolidone) and silver nanoparticles, the solution was diluted with ethanol and centrifuged at 2,000 r.p.m. for 15 min. After repeating several times until the supernatant became transparent, the solution was redispersed in H 2 O. The resulting bicrystalline [55] AgNWs were typically 100–120 nm in diameter and 3–10 μm in length, as determined by scanning electron microscopy. Finite different time domain simulation Simulations were performed using the Lumerical FDTD Solutions software package ( http://www.lumerical.com ). A 4-μm-long AgNW with 100 nm diameter was simulated surrounded by a background index of 1.4, which corresponds to the index of refraction for PDMS. The QD fluid was assumed to have the same index. Simulations were performed by exciting the AgNW with a transient dipole source, and calculating the field after the dipole excitation had finished. How to cite this article : Ropp, C. et al. Nanoscale imaging and spontaneous emission control with a single nano-positioned quantum dot. Nat. Commun. 4:1447 doi: 10.1038/ncomms2477 (2013).